Engineering interlocking DNA rings with weak physical interactions Catenanes are intriguing molecular assemblies for engineering unique molecular devices. The resident rings of a catenane are expected to execute unhindered rotation around each other, and to do so, they must have weak physical interactions with each other. Due to sequence programmability, DNA has become a popular material for nanoscale object engineering. However, current DNA catenanes, particularly in the single-stranded (ss) form, are synthesized through the formation of a linking duplex, which makes them less ideal as mobile elements for molecular machines. Herein we adopt a random library approach to engineer ssDNA [2] catenanes (two interlocked DNA rings) without a linking duplex. Results from DNA hybridization, double-stranded catenane synthesis and rolling circle amplification experiments signify that representative catenanes have weak physical interactions and are capable of operating as independent units. Our findings lay the foundation for exploring free-functioning interlocked DNA rings for the design of elaborate nanoscale machines based on DNA. Nature makes use of intricate molecular motors to execute complex mechanical motions that drive important cellular activities such as molecular trafficking and muscle contraction [1] . Rotary motors can carry out molecular motions using nanoscale shafts and bearings, and linear motors can make step-by-step movements along molecular tracks [2] . These elegant systems have inspired attempts to create synthetic molecular motors that are capable of performing controlled mechanical operations such as unidirectional rotary motion and bidirectional circumrotation [3] , [4] , [5] , [6] , [7] . Synthetic molecular motors are often designed to contain two or more mechanically interlocked macrocycles (molecular assemblies also known as catenanes) [8] . Catenanes represent a highly unique class of molecular architectures as their component rings are held together not by any chemical or physical bond, but by a ‘mechanical bond’ that is unavailable in conventional molecular assemblies [9] . A distinct outcome of such an arrangement is that the component rings in a catenane are able to rotate freely around each other [8] , [9] . Many synthetic catenanes have been prepared from organic building blocks and exploited as primitive molecular devices such as positional switches and nanomotors [6] , [7] , [10] , [11] , [12] , [13] . DNA, due to its sequence programmability, biocompatibility and ease of manipulation, has become a popular polymeric system for the design of nanoobjects in recent years [14] . DNA has been used to construct an increasing number of topologically interesting nanostructures [15] , [16] , [17] , [18] , [19] , [20] , [21] , [22] , [23] , [24] , [25] . For example, Willner and co-workers [21] have successfully designed DNA [2] and [3] catenanes and exploited a simple strand-displacement strategy to program directional reconfiguration of DNA catenane topologies. Most of the currently reported interlocked nanoobjects, however, are created from linear single-stranded (ss) DNA molecules via DNA–DNA hybridization, followed by ring closures. Because of this, the individual components in these catenanes are physically engaged via a double-stranded (ds) region made of one or more helical turns. The existence of such a strong linking duplex prevents component rings from moving or rotating independently. Those catenanes cannot be used as free-functioning components for molecular machines. Schmidt and Heckel have reported an interesting approach for preparing DNA catenanes [23] . Instead of preparing ss catenanes, they opted to synthesize ds catenanes through the closure of two C-shaped dsDNA fragments linked together via two temperature-sensitive chemical linkages. Resolution of the chemical cross-linkers at an elevated temperature allows the two-component ds rings to function independently. The two key factors that empower this method are the design of DNA fragments with a C-curvature and the choice of the chemical cross-linkers that can position the two C-fragments in catenation-permissible orientation before ring closure. In another report, Li and his co-workers [25] have employed a recombinase to convert a dsDNA ring that contains two recombination-recognition sites into two interlocked dsDNA rings. Both methods, however, have yet to be applied for the synthesis of ssDNA catenanes. Catenanes made of ssDNA rings can offer some unique advantages over the ds counterparts. These include the incorporation of functional moieties (that is, DNAzymes and DNA aptamers) and the loading of additional DNA molecules through DNA–DNA hybridization. Here, we develop a strategy that is capable of efficiently producing ss catenanes without the use of a linking duplex so that each component ring still has the flexibility to function independently. This is not a trivial matter because DNA molecules to be catenated have to interact somehow. We take advantage of in vitro selection, which uses iterative cycles of selection and amplification to search for functional DNA or RNA molecules from a synthetic DNA or RNA pool containing 10 13 –10 16 different sequence variants [26] , [27] . By this approach, we isolate many sequences from a random DNA pool that can form DNA [2] catenanes (two interlocked DNA rings) with a premade ssDNA circle. From several characterization experiments, we conclude that the component rings within these catenanes do not have strong physical engagement and have excellent capability to function independently. DNA catenation method design Two methods, illustrated as A and B in Fig. 1 , have been reported for preparing a DNA [2] catenane (simplified as D2C in this work, which refers to two interlocked DNA rings) [15] , [16] , [19] . Method A uses a premade circular DNA, denoted here as C DNA i , and a linear DNA, L DNA ii , and their sequences are specifically designed such that the 5′ and 3′ ends of L DNA ii can juxtapose on C DNA i for ring closure by DNA ligase. Method B is similar, except that the hybridization between C DNA i and L DNA ii occurs within the central segment of L DNA ii and a separate DNA molecule is used to engage the ends of L DNA ii for ring closure. Both methods lead to production of a D2C that is physically bonded by a strong linking duplex [28] , [29] . In addition, the sequences of DNA i and DNA ii have to be carefully designed to eliminate complicating secondary structures and to maximize catenation yield [28] . 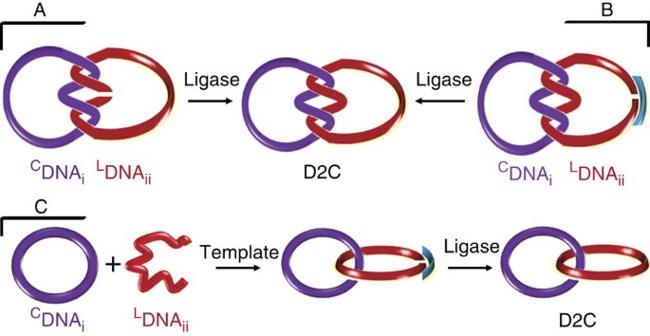Figure 1: Strategies for preparing D2Cs. (A) The circular DNACDNAi(purple) is used as a template upon which the two termini of the linear DNALDNAii(red) hybridize, followed by T4 DNA ligase-mediated ligation. (B) The central region ofLDNAiihybridizes withCDNAi, followed by hybridization of the two termini ofLDNAiiover a template DNA (blue), and by T4 DNA ligase-mediated ligation. Both methods A and B use predesigned DNA sequences. (C) A variation of method B.LDNAiiis designed to have a central random sequence region so that some of its members can find a way to interact withCDNAibefore template directed ring closure by T4 DNA ligase.In vitroselection is then carried out to isolate these members. Figure 1: Strategies for preparing D2Cs. (A) The circular DNA C DNA i (purple) is used as a template upon which the two termini of the linear DNA L DNA ii (red) hybridize, followed by T4 DNA ligase-mediated ligation. (B) The central region of L DNA ii hybridizes with C DNA i , followed by hybridization of the two termini of L DNA ii over a template DNA (blue), and by T4 DNA ligase-mediated ligation. Both methods A and B use predesigned DNA sequences. (C) A variation of method B. L DNA ii is designed to have a central random sequence region so that some of its members can find a way to interact with C DNA i before template directed ring closure by T4 DNA ligase. In vitro selection is then carried out to isolate these members. Full size image We sought to minimize the physical engagement by exploring a random library approach, illustrated as method C in Fig. 1 . It represents an expansion of method B; however, instead of using a defined L DNA ii sequence, an L DNA ii library is employed. The library is generated via randomization of the central region of L DNA ii . With the use of such a DNA library, in vitro selection can then be carried out to search for DNA molecules that can catenate efficiently with C DNA i . More importantly, we hypothesize this method can lead to the discovery of L DNA ii sequences that can form D2C without using an extensive linking duplex and thus the two DNA rings in the D2C are much less engaged and can act as independent units. Sequence design The sequence of L DNA i is provided in Supplementary Fig. 1 . It contains 90 nucleotides (nt) and an embedded Bam HI restriction enzyme recognition site (for facilitating D2C characterization later). L DNA i can be circularized into C DNA i using the 24-nt oligonucleotide T DNA i ( Supplementary Fig. 1 ). L DNA i and C DNA i can be easily distinguished using 10% denaturing polyacrylamide gel electrophoresis (dPAGE; Supplementary Fig. 1 ). The sequence of L DNA ii is provided in Supplementary Fig. 2a . It is 80-nt long, with 51 central random nt and an Eco RI restriction enzyme recognition site incorporated into one of two constant regions flanking the random domain. L DNA ii can be circularized into C DNA ii using T DNA ii ( Supplementary Fig. 2a ) as the ligation template and can be amplified in a polymerase chain reaction (PCR) using primers 1 and 2 ( Supplementary Fig. 2a ). In vitro selection strategy The in vitro selection strategy to isolate catenating L DNA ii sequences is illustrated in Supplementary Fig. 2b . In step I, a pool of 5′ phosphorylated L DNA ii is incubated first with C DNA i and then with T DNA ii . The two hybridization reactions need to be conducted separately because L DNA ii cannot thread through C DNA i if its two termini juxtapose onto T DNA ii first. The ring closure of L DNA ii by T4 DNA ligase is carried out in step II. The uncyclized L DNA ii are digested with an exonuclease and D2Cs are isolated by dPAGE in step III. The purified D2Cs are subject to two successive PCRs—PCR1 (step IV) uses primers P1 and P2 while PCR2 (step V) uses P1 and P3 as the primers. Since P3 is terminated with a ribonucleotide, the dsDNA amplicons contain a single ribonucleotide right in the front of L DNA ii , which is hydrolyzed by NaOH in step VI. The L DNA ii molecules in the DNA mixture is purified by dPAGE, phosphorylated at their 5′ end (step VII) and used to initiate the next round of selection (repeating steps I–VII). In vitro selection results Because we were interested in isolating L DNA ii sequences that can undergo catenation with C DNA i , for each round of selection, we measured the ‘degree of catenation’, which is defined as the amount of catenated C DNA ii over that of uncatenated C DNA ii . The results are provided in Fig. 2a . 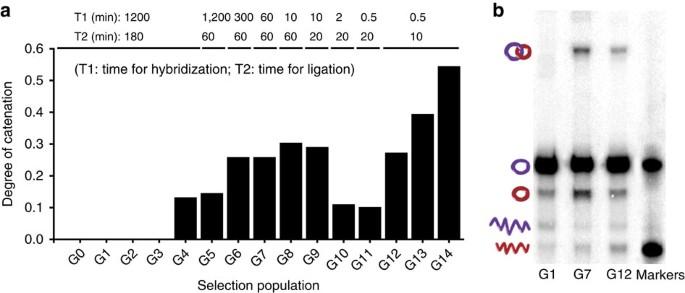Figure 2:In vitroselection of D2Cs. (a)In vitroselection progress, as measured by the degree of catenation ofLDNAiifor each selection round. T1: time allowed for the hybridization betweenCDNAiandLDNAii. T2: time for DNA ligation. (b) dPAGE analysis of G1, G7 and G12 DNA pools. Figure 2: In vitro selection of D2Cs. ( a ) In vitro selection progress, as measured by the degree of catenation of L DNA ii for each selection round. T1: time allowed for the hybridization between C DNA i and L DNA ii . T2: time for DNA ligation. ( b ) dPAGE analysis of G1, G7 and G12 DNA pools. Full size image Catenated DNA was not observed during the first four rounds (corresponding to generation 0–3, G0–G3). However, a DNA band with slower electrophoretic mobility than C DNA i appeared in G4. From round 6, two reaction parameters, T1 ( C DNA i and L DNA ii hybridization time) and T2 (DNA ligation time), that were deemed to influence the degree of catenation, were changed to isolate L DNA ii molecules that are most effective in catenating. Specifically, T1 was progressively decreased from 1,200 min (G0–G5) to 300 min (G6), 60 min (G7), 10 min (G8 and G9), 2 min (G10) and finally, 0.5 min (G11–14); T2 was reduced from 180 min (G0–G4) to 60 min (G5–G8), 20 min (G9–G11), and finally, 10 min (G12–G14). Figure 2b shows dPAGE analysis of crude catenated products from G1, G7 and G12 as representative pools. By the 15th round of selection (G14), the degree of catenation increased to ~0.5 even with rather short T1 and T2. G14 was subject to cloning and sequencing to obtain the enriched L DNA ii sequences. Seventy-two DNA sequences belonging to 49 classes were obtained; four of them— L DNA ii 1, 2, 3 and 4—are shown in Fig. 3a , and the rest are provided in Supplementary Fig. 3 . The relatively large sequence diversity may reflect the fact that the random region of 51 nt in L DNA ii offers diverse ways to interact with C DNA i that has 90 nt. 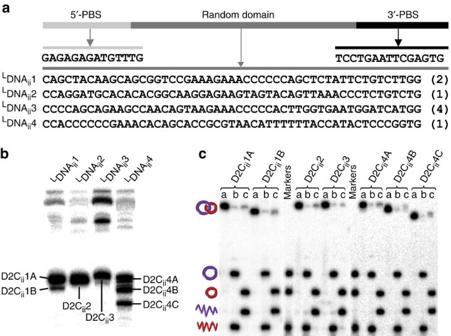Figure 3: Characterization of candidate D2Cs. (a) Four representativeLDNAiisequences derived byin vitroselection. PBS: primer-binding site. The number in the parenthesis next to each sequence represents the copy number of the sequence in the sequenced clones. (b) dPAGE analysis of ring products fromCDNAiand eachLDNAii. The suspected D2Cs are marked as D2CiiNX (N, the number given for theLDNAiisequence class; X=A, B, or C, representing sister D2Cs from the sameLDNAii). (c) Restriction digestion of all D2Cs marked inb. Each candidate D2C was incubated (a) without any restriction enzyme, (b) withEcoRI (which linearizesCDNAii) and (c) withBamHI (that digestsCDNAi). Figure 3: Characterization of candidate D2Cs. ( a ) Four representative L DNA ii sequences derived by in vitro selection. PBS: primer-binding site. The number in the parenthesis next to each sequence represents the copy number of the sequence in the sequenced clones. ( b ) dPAGE analysis of ring products from C DNA i and each L DNA ii . The suspected D2Cs are marked as D2C ii NX ( N , the number given for the L DNA ii sequence class; X=A, B, or C, representing sister D2Cs from the same L DNA ii ). ( c ) Restriction digestion of all D2Cs marked in b . Each candidate D2C was incubated ( a ) without any restriction enzyme, ( b ) with Eco RI (which linearizes C DNA ii ) and ( c ) with Bam HI (that digests C DNA i ). Full size image Characterization of candidate D2Cs The four L DNA ii sequences shown in Fig. 3a were examined for their ability to produce D2Cs with C DNA i . Each radioactive L DNA ii was incubated with C DNA i (also radioactive), followed by ring closure in the presence of T DNA ii and T4 DNA ligase. Uncircularized L DNA ii was degraded by T4 DNA polymerase while all circular DNA molecules remained intact as they are resistant to the exonuclease activity of the polymerase [15] . The suspected D2Cs were purified for further characterization below. Each candidate D2C is given a specific name (marked in Fig. 3b ) that reflects the identity of the L DNA ii involved (note that all D2Cs in this work contain the same C DNA i ). For example, only one candidate D2C was observed with L DNA ii 2 and we name it D2C ii 2. For L DNA ii 4, however, three different D2Cs were produced, which are named D2C ii 4A, D2C ii 4B, and D2C ii 4C, respectively. To confirm that each candidate D2C indeed contains a C DNA i and a C DNA ii , we carried out restriction digestion with Bam HI and Eco RI, which linearize C DNA i and C DNA ii , respectively, when T DNA i and T DNA ii were supplied as the template. Each digested D2C was analysed by dPAGE, and the results are depicted in Fig. 3c . Not surprisingly, each candidate D2C indeed produced two expected products upon digestion with Eco RI or Bam HI: treatment with Eco RI resulted in C DNA i and L DNA ii (lane b) while digestion with Bam HI generated C DNA ii and L DNA i (lane c). The identical cleavage product pattern observed for all seven candidate D2Cs indicates that each of them is indeed composed of one C DNA i and one C DNA ii interlocked to each other. One interesting observation is worth commenting: individual L DNA ii molecules exhibit varying catenating patterns ( Fig. 3b ). For L DNA ii 1, two different D2Cs were observed, with D2C ii 1A as the main product (87%) and D2C ii 1B (13%) as the minor product. Similarly, three D2Cs in comparable amounts were seen with L DNA ii 4 and they were D2C ii 4A (39%), D2C ii 4B (34%) and D2C ii 4C (27%). In contrast, only one D2C was observed for both L DNA ii 2 and L DNA ii 3 (named D2C ii 2 and D2C ii 3, respectively). The sister D2Cs of L DNA ii 1 and L DNA ii 4 exhibited considerable differences in gel mobility on dPAGE, which was lost upon linearization with Eco RI or Bam HI. These findings suggest that these sister D2Cs differ only in topological properties. Although deciphering these properties is beyond the scope of the current study, we believe that the sister D2C with slowest gel mobility—D2C ii 1A for L DNA ii 1 and D2C ii 4A for L DNA ii 4—has a topological cross of 1 (thus denoted one-cross D2C) while the sister D2Cs with faster gel mobility have 2 or 3 topological crosses (thus they are more compact and move faster on PAGE gels) [25] . Specifically, D2C ii 2B and D2C ii 4B have two topological crosses while D2C ii 4C has three topological crosses. We also analysed 5 more L DNA ii sequences for the ability to form D2Cs with C DNA i , and the results are shown in Supplementary Fig. 4 . L DNA ii 5 and L DNA ii 9 produced a single D2C while L DNA ii 6, L DNA ii 7 and L DNA ii 8 generated 2 or 3 sister D2Cs. Examining one-cross D2Cs for DNA–DNA hybridization Strikingly, all nine DNA ii sequences examined so far either produced a single one-cross D2C or generated a one-cross D2C as the main product, which represents the desirable catenane candidates where two DNA rings have weak physical interactions and are thus capable of functioning as independent units. We first investigated the sequence availability of each DNA ring in representative D2Cs for hybridization with DNA oligonucletides with complementary sequences. We examined D2C ii 2, D2C ii 3 and D2C ii 4A for this purpose. Four complementary oligonucleotides (CO) were designed for each C DNA ii —the CO set for C DNA ii 3, named CO ii 3.1–4, is shown in Fig. 4a and those for C DNA ii 2 and C DNA ii 4 are provided in Supplementary Fig. 5 . Similarly, five COs were designed for C DNA i , which are named CO i .1–5 accordingly ( Fig. 4b ). 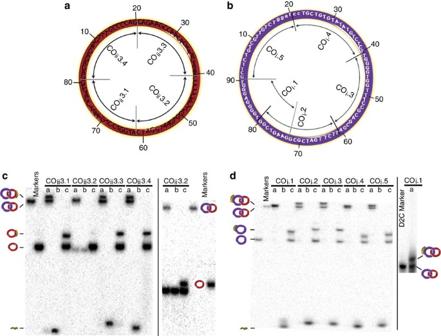Figure 4: Sequence availability of D2Cii3 for DNA hybridization. (a) COs designed forCDNAii3, which are named COii3.1–4. (b) COs, named COi.1–5, designed forCDNAi. (c) nPAGE analysis of COii3–D2Cii3 mixtures. A longer nPAGE was conducted for COii3.2/D2Cii3 to achieve better resolution of DNA bands. (d) nPAGE analysis of COi–D2Cii3 mixtures. For each CO, three samples were analysed: lane a, CO-D2C mixture; lane b, CO alone; lane c, CO-CDNA mixture. A longer nPAGE was conducted for COi.1/D2Cii3 to achieve better resolution of DNA bands. Figure 4: Sequence availability of D2C ii 3 for DNA hybridization. ( a ) COs designed for C DNA ii 3, which are named CO ii 3.1–4. ( b ) COs, named CO i .1–5, designed for C DNA i . ( c ) nPAGE analysis of CO ii 3–D2C ii 3 mixtures. A longer nPAGE was conducted for CO ii 3.2/D2C ii 3 to achieve better resolution of DNA bands. ( d ) nPAGE analysis of CO i –D2C ii 3 mixtures. For each CO, three samples were analysed: lane a, CO-D2C mixture; lane b, CO alone; lane c, CO- C DNA mixture. A longer nPAGE was conducted for CO i .1/D2C ii 3 to achieve better resolution of DNA bands. Full size image Each CO was allowed to hybridize with a relevant C DNA or D2C, and the DNA mixture was subjected to 10% nondenaturing polyacrylamide gel electrophoresis (nPAGE). The hybridization results for D2C ii 3 are shown in Fig. 4 while those for D2C ii 2 and D2C ii 4A are provided in Supplementary Fig. 5 . For each CO, three samples were analysed: CO alone (lane b), CO with the matching C DNA (lane c) and CO with the matching D2C (lane a). It should be noted that each CO was set as the limiting reagent so that double bands could be observed for a given C DNA or its D2C (this was done mainly because we found it was harder to determine the absolute positions of a given D2C and its CO hybrid on nPAGE). Double bands were observed when each CO i was incubated with either C DNA i or each D2C ( Fig. 4d ; Supplementary Fig. 5c,f ), along with the disappearance of the CO i band. It should be noted that a longer running time was needed to resolve the CO i .1-D2C hybrid from D2C itself (comparing the lane ‘a’ under ‘CO i .1’ in the main gel in Fig. 4d with the same lane in the supplemental gel shown on the right of Fig. 4d ). These results indicate that each targeted sequence element of C DNA i within a given D2C is indeed available for hybridization. The same observation was made for the entire CO ii 4 set ( Supplementary Fig. 5e ), three out of four within the CO ii 3 set ( Fig. 4c ) and two out of four within the CO ii 2 set ( Supplementary Fig. 5b ). The exceptions are CO ii 3.2, CO ii 2.2, and CO ii 2.3. However, upon careful analysis of the experimental results, it was found that the lack of hybridization in each case was simply a reflection of possibly the secondary structure of a particular CO or C DNA itself rather than the D2C. In the case of CO ii 3.2, it appears that it forms a higher-order structure that has a gel mobility just below that of C DNA ii 3 (see the last three lanes of Fig. 4c ). Because CO ii 3.2 contains five consecutive G residues at its 5′ end, we suspect that the corresponding DNA band on nPAGE represents a stable guanine quadruplex species, which makes CO ii 3.2 unavailable for hybridization with either C DNA ii 3 or D2C ii 3. However, no higher-order DNA species was observed for both CO ii 2.2 and CO ii 2.3, and sequence inspection of these two oligonucleotides did not reveal any strong secondary structure. Thus the lack of hybridization does not appear to be a property of the concerned CO. In addition, it was observed that each CO was unable to hybridize to both C DNA ii 2 and D2C ii 2. Based on these analyses, we attribute the lack of hybridization to the existence of strong secondary or tertiary structural interactions at the CO ii 2.2 and CO ii 2.3-binding sites within C DNA ii 2, which make these two sequence elements unavailable for hybridization. More importantly, we can conclude that the formation of interlocking structures within all examined candidate one-cross catenanes does not alter the hybridization ability of the component C DNA i or C DNA ii . Fabrication of dsD2Cs The DNA hybridization experiment above suggests that the component C DNA i and C DNA ii within each ssD2C examined does not appear to utilize strong molecular interactions (such as extensive duplex formation) to engage each other for the formation of D2C. To further verify that this indeed is the scenario, we sought to prepare dsD2Cs and examine whether the ds rings in such dsD2Cs are truly independent. Two ssD2Cs, D2C ii 3 and D2C ii 9, were used for this investigation, and the data are presented in Fig. 5 . 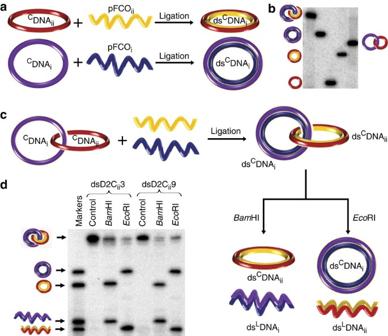Figure 5: Double-stranded D2Cs. (a) Scheme for using pFCOiand pFCOiito convert ssCDNAiand ssCDNAiiinto ds species. (b) nPAGE analysis of ssCDNAii3, dsCDNAii3, dsCDNAi, ssD2Cii3 and dsD2Cii3. (c) Scheme for preparing and characterizing dsD2C. pFCOiand pFCOiiwere allowed to hybridize with an ssD2C, followed by ligase-mediated DNA ligation. Each dsD2C was purified and digested withBamHI orEcoRI. (d) Results of restriction digestion of dsD2Cii3 and dsD2Cii9. Each dsD2C was digested withBamHI orEcoRI, and digested mixture was subject to 10% nPAGE analysis. Controls, no restriction digestion. Figure 5: Double-stranded D2Cs. ( a ) Scheme for using pFCO i and pFCO ii to convert ss C DNA i and ss C DNA ii into ds species. ( b ) nPAGE analysis of ss C DNA ii 3, ds C DNA ii 3, ds C DNA i , ssD2C ii 3 and dsD2C ii 3. ( c ) Scheme for preparing and characterizing dsD2C. pFCO i and pFCO ii were allowed to hybridize with an ssD2C, followed by ligase-mediated DNA ligation. Each dsD2C was purified and digested with Bam HI or Eco RI. ( d ) Results of restriction digestion of dsD2C ii 3 and dsD2C ii 9. Each dsD2C was digested with Bam HI or Eco RI, and digested mixture was subject to 10% nPAGE analysis. Controls, no restriction digestion. Full size image We prepared a radioactive, 5′-phosphorylated and fully complementary oligonucleotide (pFCO) that binds C DNA i , C DNA ii 3 or C DNA ii 9. Each pFCO was allowed to hybridize with C DNA i , C DNA ii 3, C DNA ii 9, ssD2C ii 3 and ssD2C ii 9, followed by ligation with T4 DNA ligase ( Fig. 5a,c ). Each ds species was purified by PAGE and subject to further characterization. First, the relative gel mobility of ss C DNA, ds C DNA, ssD2C and dsD2C was analysed ( Fig. 5b ), followed by characterization of purified dsD2Cs via digestion with Bam HI and Eco RI ( Fig. 5d ). It was predicted that if each component ds C DNA within a dsD2C underwent a weak physical engagement, the Bam HI digestion would produce a ds L DNA i and a ds C DNA ii while the Eco RI treatment would instead produce a ds L DNA ii and a ds C DNA i . Indeed, as shown in Fig. 5d , two products were produced from each restriction digestion, each of which exhibited a gel mobility that matched precisely to that of the expected ds L DNA or ds C DNA. The lack of any intermediate DNA bands on nPAGE conclusively indicates that each component ds C DNA in dsD2C ii 3 and dsD2C ii 9 does not physically interact with the other ds C DNA. Rolling circle amplification of D2Cs Next we assessed select D2Cs for independent functions, specifically their ability to function as circular templates for rolling circle amplification (RCA). Four D2Cs were examined in this section and they are D2C ii 1A, 2, 3 and 9. Following each RCA, Bam HI and Eco RI were used to digest the RCA product, which produced monomeric L DNA i or L DNA ii that can be easily analysed by dPAGE. We first conducted comparative RCA reactions to assess the efficiency of RCA, RCA-E, on a free C DNA i (or C DNA ii ) and a catenated C DNA i (or C DNA ii ). RCA-E is defined as the ratio between the amount of the RCA product obtained with the catenated C DNA with the matching free C DNA. The RCA-E was observed to be within the range of 0.9–1.2 ( Fig. 6a ), suggesting that catenation has minimal impact on the ability of either C DNA i or C DNA ii to function as the template for RCA. 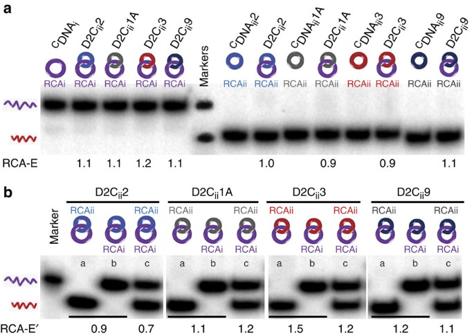Figure 6: RCA using a D2C as the template. Four different D2Cs—D2Cii1A, 2, 3 and 9—were examined. (a) RCA on one of the interlocked rings. Left panel: RCA on uncatenatedCDNAiandCDNAiin each D2C. Right panel: RCA on a given uncatenatedCDNAiiand theCDNAiiin the matching D2C. Following each RCA,BamHI andEcoRI were used to digest the RCA product, which produced monomericLDNAiorLDNAiito facilitate RCA efficiency comparison by dPAGE analysis. RCA-E=(amount of RCA product from catenatedCDNAiorii)/(amount of RCA product from uncatenatedCDNAiorii). (b) Concurrent RCA on both interlocked rings. For each D2C, separate RCA onCDNAi(lane b) andCDNAii(lane a) as well as concurrent RCA on both (lane c) were performed. RCA-E′=(amount of RCA product fromCDNAiin a given D2C)/(amount of RCA product fromCDNAiiin the same D2C). Figure 6: RCA using a D2C as the template. Four different D2Cs—D2C ii 1A, 2, 3 and 9—were examined. ( a ) RCA on one of the interlocked rings. Left panel: RCA on uncatenated C DNA i and C DNA i in each D2C. Right panel: RCA on a given uncatenated C DNA ii and the C DNA ii in the matching D2C. Following each RCA, Bam HI and Eco RI were used to digest the RCA product, which produced monomeric L DNA i or L DNA ii to facilitate RCA efficiency comparison by dPAGE analysis. RCA-E=(amount of RCA product from catenated C DNA i or ii )/(amount of RCA product from uncatenated C DNA i or ii ). ( b ) Concurrent RCA on both interlocked rings. For each D2C, separate RCA on C DNA i (lane b) and C DNA ii (lane a) as well as concurrent RCA on both (lane c) were performed. RCA-E′=(amount of RCA product from C DNA i in a given D2C)/(amount of RCA product from C DNA ii in the same D2C). Full size image We next tested each D2C for its ability to undergo concurrent RCA reactions where each catenated C DNA was simultaneously exploited as the template. As the results in Fig. 6b have shown, the double RCA with each D2C, followed by restriction digestion, indeed produced two monomers that are identical to the monomers obtained with each single RCA. Furthermore, we also measured the relative RCA efficiency, RCA-E′, defined as the ratio between the amount of the RCA product from C DNA i and that from C DNA ii within the same D2C. Comparable RCA-E′ values were observed for both the double RCA reactions and two separate RCA reactions when the same D2C was used. Taken together, these results illustrate that the component C DNAs within the examined D2Cs can indeed function as independent units. Independent and cooperative functions of D2Cs Finally, we investigated some potential applications of the weakly interacting interlocked ss rings. First, we assessed whether we could carry out two independent functions with D2Cs: DNA hybridization on one ring and RCA on another. D2C ii 1A, 3 and 9 were examined in this experiment and the data are provided in Fig. 7a (D2C ii 1A) and Supplementary Fig. 6 (D2C ii 3 and 9). Each D2C was allowed to hybridize with one of the two DNA probes, DP i and DP ii (which hybridize with C DNA i and C DNA ii , respectively), as well as biotinated or biotin–streptavidin tagged versions, followed by the RCA reaction on the free DNA ring. The RCA efficiency data presented in Fig. 7a and Supplementary Fig. 6 indicate that the hybridization with these DNA or DNA protein molecules on one ring had little effect on the RCA reaction of the other ring. 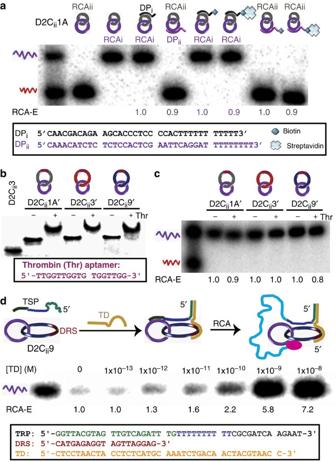Figure 7: Potential utilities of D2Cs. (a) Independent RCA and DNA hybridization on D2Cii1A. Lane 1:LDNAiandLDNAiimarkers; lanes 2, 5, 8 and 9: RCA on catenatedCDNAiiwhileCDNAicarried no DP1, DPi, biotinated DPiand biotin–streptavidin tagged DPi; lanes 3, 4, 6 and 7: RCA on catenatedCDNAiwhileCDNAiicarried no DPii, DPii, biotinated DPiiand biotin–streptavidin tagged DPii. (b) Thr-binding assay involving three D2Cs modified with a Thr aptamer domain. (c) Independent RCA and Thr binding on aptamer-containing D2Cs. (d) Use of D2C for DNA detection.CDNAiiof D2Cii9 was expanded to contain a DRS. A target-specific primer (TSP) was also designed. In the presence of a TD of interest, TSP, DRS and D2C assemble, which enables RCA. Fora,candd, following RCA,BamHI andEcoRI were used to digest the RCA product, which produced monomericLDNAiorLDNAiito facilitate RCA efficiency comparison with dPAGE analysis. RCA-E=(amount of RCA product from the test RCA)/(amount of RCA product from the control RCA). Pink oval: phi29 DNA polymerase. Figure 7: Potential utilities of D2Cs. ( a ) Independent RCA and DNA hybridization on D2C ii 1A. Lane 1: L DNA i and L DNA ii markers; lanes 2, 5, 8 and 9: RCA on catenated C DNA ii while C DNA i carried no DP1, DP i , biotinated DP i and biotin–streptavidin tagged DP i ; lanes 3, 4, 6 and 7: RCA on catenated C DNA i while C DNA ii carried no DP ii , DP ii , biotinated DP ii and biotin–streptavidin tagged DP ii . ( b ) Thr-binding assay involving three D2Cs modified with a Thr aptamer domain. ( c ) Independent RCA and Thr binding on aptamer-containing D2Cs. ( d ) Use of D2C for DNA detection. C DNA ii of D2C ii 9 was expanded to contain a DRS. A target-specific primer (TSP) was also designed. In the presence of a TD of interest, TSP, DRS and D2C assemble, which enables RCA. For a , c and d , following RCA, Bam HI and Eco RI were used to digest the RCA product, which produced monomeric L DNA i or L DNA ii to facilitate RCA efficiency comparison with dPAGE analysis. RCA-E=(amount of RCA product from the test RCA)/(amount of RCA product from the control RCA). Pink oval: phi29 DNA polymerase. Full size image The second experiment concerns the incorporation of a DNA aptamer sequence into one of the resident rings of D2Cs and the assessment of the influence of the aptamer target binding on the RCA over the second ring. We chose the well-known human thrombin (Thr)-binding DNA aptamer [30] for the incorporation into C DNA ii of the following three catenanes: D2C ii 1A, 3 and 9. The synthetic scheme and the relevant DNA sequences are provided in Supplementary Fig. 7 . The nPAGE analysis provided in Fig. 7b shows that the aptamer-containing D2Cs retain the ability to bind its cognate target as each D2C exhibited a much-reduced gel mobility in the presence of Thr. More importantly, as seen with the data shown in Fig. 7c , the binding of Thr to the aptamer within the modified C DNA ii in each D2C did not significantly affect the efficiency of RCA on the interlocked C DNA i . The final experiment involves the use of a modified D2C for DNA detection, as illustrated in Fig. 7d . A DNA recognition sequence (DRS) was inserted into the C DNA ii of D2C ii 9, which can bind to part of a target DNA (TD) sequence. A target-specific primer was also designed in which its 3′ end can bind C DNA i and act as the RCA primer but its 5′ end can recognize part of TD. This design utilizes one of the interlocked rings for target recognition and the other ring for signal amplification. Such a system can indeed achieve target-dependent RCA and was able to detect low pM concentrations of the DNA target ( Fig. 7d ). Yield of preparation One important factor for consideration when making DNA nanodevice is the preparation yield [28] , [31] . Since D2Cs produced in our approach do not appear to be based on extensive base-pairing interactions, their preparation may suffer from lower reaction yield. For this consideration, we examined the yield of D2C with three selected L DNA ii sequences: L DNA ii 2, L DNA ii 3 and L DNA ii 9. For this experiment, radioactive (*) C DNA i was allowed to undergo catenation with each non-radioactive L DNA ii and the D2C yield is calculated as *D2C/(*D2C+ * C DNA i ). By this method, we found that the catenation yield of L DNA ii 1, L DNA ii 3 and L DNA ii 9 is 34, 73 and 59%, respectively ( Supplementary Fig. 8 ). Using in vitro selection, we have derived many ssDNA molecules that are capable of threading through a premade DNA ring to allow for the synthesis of ssD2Cs. Most of the examined DNA sequences generate a single ssD2C with one topological cross while a selective few can produce 2–3 sister ssD2Cs with 1, 2 or 3 topological crosses. We did not take any special measures during in vitro selection to exclude interlocking by hybridization as we hypothesized that there are abundant sequences in a DNA pool capable of binding a premade ssDNA ring via molecular interactions that are not based on a long stretch of base pairs. From the comparative hybridization experiment using a set of CO that target each component ring for binding, it is clear that the hybridization ability of each component ring in separation is preserved after catenation. From this observation, we were able to make dsD2Cs simply through ssD2C-templated ligation of two oligonucleotides fully complementary to the component ssDNA rings. Restriction digestion followed by nPAGE analysis resulted in clearly separated L DNA and C DNA pairs, indicating that two-component dsDNA rings in dsD2Cs do not have strong physical engagement beyond the topological companionship. This result in turn can serve as the evidence to support our proposition that the interlocking ssDNA rings in the original ssD2Cs engage each other not through strong component–component interactions but through weak physical interactions (otherwise each dsD2C would be comprised of partially complementary DNA rings with cross-pairing bubble regions, which would not produce clearly separated L DNA and C DNA pairs on nPAGE). The lack of strong physical engagement is further supported by the results from the RCA experiments, which show that the efficiency of RCA over catenated ssDNA ring template is equal to that over free ssDNA ring template. Although the resident rings in the examined interlocked DNA structures do not appear to have strong physical engagement, they must interact somehow. These molecular interactions certainly enabled the selection of winning sequences from the random sequence pool and were also the basis for the observed high synthesis yields. One possible scenario is that the selected sequences might have explored a combination of tertiary and base-pairing interactions to achieve relatively loose physical grip with the premade ring structure. Deciphering these underlining molecular interactions will constitute a future research interest. Interlocked ssDNA rings with weak physical interactions represent a unique class of molecular assemblies that can be explored to achieve some intricate functions within a single molecular structure. For example, we have shown that the in vitro selected D2Cs can be further modified to enable two independent functions within one system, such as DNA hybridization and RCA, or aptamer binding and RCA. These DNA catenanes can also be used to deliver two cooperative functions, such as DNA binding-triggered signal amplification. Such 2-in-1 functions are difficult to achieve simply with a linear ssDNA molecule, particularly when one of the functions is the signal amplification. We believe the findings presented in this study lay the foundation for the future exploration of free-functioning interlocked DNA ring structures for the design of elaborate nanomachines based on DNA. Oligonucleotides and chemical reagents DNA oligonucleotides were prepared using standard phosphoramidite chemistry (W. M. Keck Facility, Yale University, New Haven, CT, USA; and Integrated DNA Technologies, Coralville, IA, USA). The random DNA library for in vitro selection was synthesized using an equimolar mixture of the four standard phosphoramidites. Each oligonucleotide was purified by 10% (8 M urea) dPAGE, and its concentration was determined spectroscopically. Deoxynucleoside 5′-triphosphates (dNTPs), T4 DNA ligase, φ29 DNA polymerase, T4 polynucleotide kinase (PNK), Taq DNA polymerase, Bam HI and Eco RI (with the matching buffer for each enzyme) were purchased from Thermo Scientific (Ottawa, ON, Canada). [α- 32 P]deoxy-GTP and [γ- 32 P]ATP were acquired from Perkin Elmer (Woodbridge, ON, Canada). All other chemicals were obtained from Sigma-Aldrich (Oakville, ON, Canada). DNA phosphorylation with [α- 32 P]ATP and PNK Radioactive DNA molecules were prepared by labelling at the 5′ terminus with [α- 32 P]ATP with the aid of PNK according to the manufacturer-supplied protocol. To ensure that all DNA molecules contain the 5′ phosphate required for ligation, PNK mediated end-labelling solution (100 μl) containing 10 μCi [α- 32 P]ATP was further incubated with 5 mM non-radioactive ATP at 37 °C for 30 min. Then, the reaction was quenched by heating the mixture at 90 °C for 5 min. The phosphorylated DNA was purified by dPAGE. Preparation of C DNA i C DNA i was prepared with 0.4 μM L DNA i and 0.48 μM T DNA i . The L DNA i and T DNA i mixture (2,690 μl) was heated at 90 °C for 1 min and cooled to room temperature. Then, 300 μl of 10 × T4 DNA ligase buffer (MBI Fermentas) was added. This was followed by addition of 10 μl of T4 DNA ligase (5 U μl −1 ; U, units) and incubation at room temperature for ~16 h. DNA in the mixture was concentrated by ethanol precipitation. After exonuclease digestion using T4 DNA polymerase (see below), C DNA i molecules were purified by dPAGE. Purified C DNA i was dissolved in water and its concentration was measured spectroscopically. Exonuclease digestion by T4 DNA polymerase C DNA (in 7 μl of water) was mixed with 2 μl of 5 × polymerase buffer [335 mM Tris–HCl, pH 8.8 at 25 °C, 33 mM MgCl 2 , 5 mM DTT, 84 mM (NH 4 ) 2 SO 4 ], followed by addition of 1 μl of T4 DNA polymerase (5 U μl −1 ). After incubation at 37 °C for 16 h, the digestion products were analysed by dPAGE. In vitro selection The initial round was performed in a volume of 120 μl under the following conditions: 0.45 μM each of 5′-phosphorylated L DNA ii , C DNA i , T DNA ii and 40 U of T4 DNA ligase. Before the ligation, the mixture of L DNA ii and C DNA i was heated at 90 °C for 1 min and cooled to room temperature. After the addition of 10 × T4 DNA ligase buffer (one tenth of the final volume), the mixture was allowed to incubate at room temperature for 20 h. Then, T4 DNA ligase and T DNA ii were added, and the ligation reaction was allowed to proceed at room temperature for 3 h. Following heat inactivation of the ligase at 90 °C for 5 min, the DNAs were concentrated by ethanol precipitation and exposed to 5 U of T4 DNA polymerase for 1 h to digest uncircularized L DNA ii . Thus treated DNA mixture was subjected to dPAGE and the gel zone corresponding to D2Cs were excised. The DNA was then eluted and used for the two PCR steps below. In PCR1, a reaction solution (50 μl) was prepared to contain the DNA prepared above, 1 μM each of P1 and P2, 200 μM each of dNTPs (dATP, dCTP, dGTP and dTTP), 1 × PCR buffer [75 mM Tris–HCl, pH 9.0, 2 mM MgCl 2 , 50 mM KCl, 20 mM (NH 4 ) 2 SO 4 ] and 5 U of Taq DNA polymerase. The mixture was first heated at 94 °C for 1 min, followed by 13 circles of 94 °C (30 s), 50 °C (45 s), 72 °C (45 s) and by 72 °C for 1 min. A small aliquot (1 μl) of the PCR1 product above was used as a template for PCR2, which was identical to PCR1 except for the replacement of P1 with the ribonucleotide terminated primer P3, the decrease of dGTP concentration to 20 μM and the inclusion of 10 μCi of [α- 32 P]dGTP as a radiolabel. The DNA product generated in PCR2 was recovered by ethanol precipitation, suspended in 90 μl of 0.25 M NaOH. The resulting solution was incubated at 90 °C for 10 min to cleave the RNA linkage introduced by P3. The cleavage solution was neutralized by the addition of 10 μl of 3 M NaOAc (pH 5.2 at 23 °C). The newly generated 86-nt ssDNA fragments were recovered by ethanol precipitation and purified by dPAGE. The purified DNA was phosphorylated at the 5′-end using PNK and ATP, followed by ethanol precipitation. The phosphorylated DNA was used for the next round of selection after spectroscopic quantification. A total of 15 rounds of selection and amplification were carried out using a similar procedure as described for the first round. However, from the sixth round, the C DNA i – L DNA ii hybridization time, T1, and the DNA ligation time, T2, were shortened as follows: round 6, T1=1,200 min and T2=60 min; round 7, T1=300 min and T2=60 min; round 8, T1=60 min and T2=60 min; round 9, T1=10 min and T2=60 min; round 10, T1 =10 min and T2=20 min; round 11, T1=2 min and T2=20 min; round 12, T1=30 s and T2=20 min; rounds 13-15, T1=30 s and T2=10 min. DNA sequences from the 15th round were amplified by PCR and cloned by the TA cloning method as previously described [32] . Preparation of D2Cs Preparation of each D2C was performed in a volume of 120 μl under the following conditions: L DNA ii (0.48 μM) and C DNA i (0.4 μM) were heated at 90 °C for 1 min and cooled to room temperature. After the addition of 10 × T4 DNA ligase buffer (one tenth of the final volume), the mixture was allowed to incubate at room temperature for 2 h. Then, T DNA ii (0.58 μM) and T4 DNA ligase (20 U) were added, and the ligation reaction proceeded at room temperature for 2 h. This was followed by heat inactivation of the ligase at 90 °C for 5 min. The DNAs in the mixture was recovered by ethanol precipitation. Finally, exonuclease digestion of remaining L DNA ii by T4 DNA polymerase and purification by dPAGE was performed, generating D2C for further analysis. Restriction digestion of D2Cs T DNA i and T DNA ii were used as the respective template for the digestion of each D2C with Bam HI and Eco RI. The mixture (8 μl) of a given D2C and T DNA (in 10-fold excess) was heated at 90 °C for 1 min, and then cooled to room temperature. After the addition of 10 × digestion buffer (supplied by Thermo Scientific) and 1 μl of the restriction enzyme (FastDigest Bam HI and Eco RI from Thermo Scientific), the resulting mixture was incubated at 37 °C for 1 h. The restriction digestion was quenched with an equal volume of the 2 × dPAGE loading buffer. The resulting solution was used for dPAGE analysis. Construction of ds C DNAs and dsD2Cs A given C DNA (0.5 μM) or D2C (0.5 μM) and a relevant pFCO (0.6 μM) were mixed, followed by the addition of 10 × T4 DNA ligase buffer (one tenth of final volume). After heating at 90 °C for 3 min, the mixture was allowed to be cooled to room temperature and incubate for 60 min. The ligation reaction was initiated by the injection of T4 DNA ligase (the final concentration=0.1 U μl −1 ). The ligation was allowed to proceed at room temperature for 2 h and then quenched by heating at 90 °C for 5 min. After ethanol precipitation, the resulting products were dissolved in water, treated with T4 DNA polymerase as described above. The resulting ds species was purified by dPAGE. RCA of C DNAs and D2Cs RCA reactions were performed in 50 μl. A 1 μl droplet of [α- 32 P]dGTP (5 μCi) was added to 43.5 μl of a reaction solution containing ~1 pmol of a given C DNA or D2C, 2 pmol of primer, 1 nmol of dGTP and 10 nmol of dATP, dTTP and dCTP. After heating at 90 °C for 5 min, the solution was cooled to room temperature for 12 min. Then, 5 μl of 10 × RCA buffer (330 mM Tris acetate, pH 7.9 at 37 °C, 100 mM magnesium acetate, 660 mM potassium acetate, 1% (v/v) Tween 20, 10 mM DTT, provided by Thermo Scientific) was added. Subsequently, 0.5 μl of φ29 DNA polymerase (10 U μl −1 ) was injected, followed by incubation at 30 °C for 10 h. Finally, the mixture was heated to 65 °C for 10 min to stop the reaction. From the reaction mixture, 1 μl was taken for restriction digestion and dPAGE analysis. Great care was taken to ensure the concentration of a given D2C and its related C DNA was the same. For example, when investigating the RCA efficiency of C DNA i , D2C ii 1, D2C ii 2, D2C ii 3 and D2C ii 4, only C DNA i was radioactively labelled so that each circular DNA template can be normalized to the same concentration using radioactivity. Independent RCA and hybridization The hybridization-RCA reaction was performed in 50 μl. Each DP (DP i or DP ii or biotinated versions, 10 pmol; no DP in controls; 15 pmol streptavidin for samples involving streptavidin) was mixed with a given D2C (0.6 pmol), [α- 32 P]dGTP (1 μCi), primer (30 pmol), dGTP (1 nmol) and dATP, dTTP and dCTP (10 nmol each), and 1 × RCA buffer. After heating at 90 °C for 5 min, the solution was cooled to room temperature for 10 min. Subsequently, 0.5 μl of φ29 DNA polymerase (10 U μl −1 ) was added, followed by incubation at 30 °C for 60 min. Finally, the mixture was heated to 65 °C for 10 min to deactivate the polymerase. From the reaction mixture, 0.5 μl was taken for restriction digestion and dPAGE analysis. Preparation of modified D2Cs The procedure for preparing Thr aptamer-bearing D2Cs is very similar to that for the preparation of regular D2Cs described above. C DNA i (0.4 μM), L DNA ii (0.48 μM), Thr aptamer (0.70 μM) and Thr template (0.58 μM) were mixed and subject to ligase-mediated ligation and dPAGE purification. DRS-containing D2C ii 9 was prepared in the same way except that DRS replaced the Thr aptamer and DRS template (5′-CAAAC ATCTC TCTCC TCCTA ACTAC CTCTC ATGCA CTCGA ATTCA GGA-3′) was used as the ligation template. Thr-binding assay This reaction was carried out in 10 μl. Thr (5 μM) and a relevant D2C (0.5 μM) was incubated at 4 °C for 30 min in the presence of 1 × T4 DNA ligase buffer before analysis of Thr–D2C complexes by nPAGE conducted at 4 °C. Independent RCA and Thr binding RCAs on C DNA i of D2C′s in the presence of Thr were carried out under the same conditions described above for ‘Independent RCA and hybridization’ except that 5 pmol of Thr were used instead of DP. DNA detection using D2C ii 9 DRS The RCA reaction was conducted as shown in Independent RCA and hybridization except for the following: (1) the catenane was D2C ii 9 DRS (10 nM); (2) the primer was target-specific primer (50 nM) and (3) the TD was used at 0, 0.0001, 0.001, 0.01, 0.1, 1 and 10 nM. Reaction yield assessment Non-radioactive phosphorylated L DNA ii (11.2 μl, 13.0 μM) and radioactive C DNA i (4.3 μl, 16.8 μM) were added to 232 μl of water. The mixture was heated at 90 °C for 3 min, followed by cooling to room temperature for 10 min. Then, 30 μl of 10 × T4 DNA ligase buffer was added and the mixture was incubated at room temperature for 120 min before the addition of 16.8 μl of T DNA ii (10.6 μM) and 5 μl of T4 DNA ligase (5 U μl −1 ) followed by incubation at room temperature for 120 min. Subsequently, the DNA mixture was heated at 90 °C for 5 min and cooled to room temperature. The DNA was then concentrated by ethanol precipitation. After exposure to T4 DNA polymerase (to digest the uncyclized L DNA ii ), the yield of D2C from each L DNA ii was evaluated by dPAGE. How to cite this article : Wu, Z.-S. et al. Engineering interlocking DNA rings with weak physical interactions. Nat. Commun. 5:4279 doi: 10.1038/ncomms5279 (2014).